Cytoplasmic parafibromin/hCdc73 targets and destabilizes p53 mRNA to control p53-mediated apoptosis The parafibromin/hCdc73 is a component of the PAFc, which controls RNA polymerase II-mediated general transcription. In parathyroid carcinoma and familial autosomal dominant hyperparathyroidism-jaw tumour (HPT-JT), hCdc73 mutations are heavily implicated, yet the underlying mechanism of its carcinogenic action is poorly understood. Here we demonstrate that hCdc73 specifically controls messenger RNA stability of p53 and p53-mediated apoptosis. hCdc73 is associated with mature p53 mRNA in the cytoplasm and facilitates its degradation. Cytoplasmic hCdc73 physically interacts with eEF1Bγ and hSki8, and this interaction is required to bind and destabilize p53 mRNA. Furthermore, enhanced association of p53 mRNA with a cancer-driven hCdc73(K34Q) mutant was also observed. As a result, reduced p53 expression as well as enhanced cell proliferation was acquired in the hCdc73 (K34Q)-overexpressed cells. Altogether, our findings indicate that hCdc73 directly targets p53 mRNA to repress p53 expression, and aberrant regulation of this interaction may lead to tumour progression. The p53 transcription factor regulates the cell cycle, apoptosis, senescence and metabolism in response to various intrinsic and extrinsic stress signals [1] , [2] . Reflecting its central role, p53 mutation or dysfunction is closely associated with the susceptibility to cancer and to malignant tumour progression [3] , [4] . p53 activity is controlled by refined, yet extremely complicated, regulatory networks that include MDM2-mediated proteosomal degradation of p53, increased translation of p53 mRNA, sequence-specific DNA binding of p53 and de-repression of intrinsically active p53 (refs 5 , 6 ). Mature p53 mRNA is also regulated during both quiescent and stress conditions [7] , [8] . For example, one p53 target gene, Wig-1 , binds to AU-rich elements in the 3′-untranslated region (UTR) of p53 and stabilizes it [8] . However, in contrast to the extensive study of p53 protein regulation, relatively little is known about the post-transcriptional control of p53 mRNA [9] . hCdc73, also known as the parafibromin/HRPT2 tumour suppressor protein, is a component of the human RNA polymerase II-associated factor complex (PAFc), which is involved in multiple steps in general transcription [10] . The evolutionally conserved PAFc, which is composed of Paf1, Cdc73, Ctr9, Leo1 and Rtf1, facilitates transcription by associating with various transcription elongation factors and by regulating post-translational histone modification [10] , [11] , [12] . PAFc is also involved in post-transcriptional process and it is required for the recruitment of 3′-end processing factors on mRNAs and non-adenylated small nucleolar RNAs [13] , [14] . Moreover, hSki8, a component of the SKI complex involved in mRNA decay, associates with PAFc in humans [15] . PAFc abnormalities have frequently been implicated in cancer. In pancreatic cancer and cancer cell lines, the hPaf1, hCdc73 and hCtr9 genomic loci are often amplified or lost [16] , [17] . Somatic and germline mutations in the hCdc73 locus have been reported in the majority of familial autosomal dominant hyperparathyroidism-jaw tumour (HPT-JT) and sporadic parathyroid carcinoma cases [18] , [19] , [20] . In addition, loss of nuclear hCdc73 staining is observed in parathyroid carcinoma [21] . Although mCdc73/HRPT2-deficient mouse embryonic fibroblasts are prone to apoptosis [22] , changes in Cdc73 expression in cell culture exert the reverse effect on cell cycle progression and apoptosis in an SV40 large T-antigen-dependent manner [23] . These observations suggest that hCdc73 plays a central role in regulating cell growth and cell death. However, it is unclear how parafibromin/hCdc73 contributes to carcinogenesis. Here we propose that the parafibromin/hCdc73 may contribute to carcinogenesis by controlling the stability of mature p53 mRNA and p53-mediated apoptosis. p53 is required for apoptosis induced by hCdc73 silencing As has been previously reported, depleting hCdc73 in HEK293 cells induced apoptosis ( Supplementary Fig. 1a ). The effect of depleting hCdc73 on apoptosis was sensitive to cell confluence; more death was observed in confluent cells ( Supplementary Fig. 1b–d ). On the other hand, the individual knockdown of other PAFc components, such as hPaf1, hCtr9 and hLeo1 but not hSki8, did not significantly affect apoptosis ( Supplementary Fig. 1e ). This result indicates that the regulatory effect of hCdc73 on apoptosis was specific to the hCdc73 protein itself, but not specific to the PAFc complex. Consistent with this hypothesis, GST-hCdc73 overexpression was sufficient to rescue hCdc73-deficient cells from apoptosis ( Supplementary Fig. 1f ). To understand how hCdc73 controls apoptosis, the expression profile of hCdc73-deficient HEK293 cells was examined. Among the differentially expressed genes, genes related to the ‘p53 signalling pathway’ were significantly enriched ( Fig. 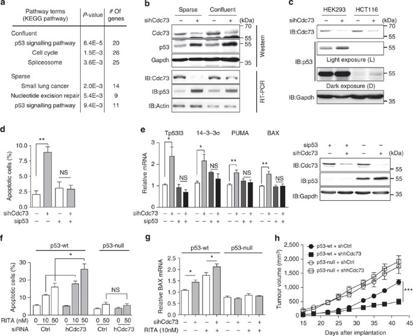Figure 1: hCdc73 controls apoptosis via p53. (a) The differential gene expression in siCtrl- versus sihCdc73-transfected HEK293 cells was analysed by microarray. Significantly affected pathways are listed. (b) HEK293 cells were transfected with siCtrl or sihCdc73, and p53 expression was analysed by western blotting (upper panel) and reverse transcriptase–PCR (RT–PCR) (bottom panel). (c) HEK293 and HCT116 cells were transfected with siCtrl or sihCdc73, and hCdc73 and p53 levels were evaluated by western blotting. (d) The apoptosis of sihCdc73- and/or sip53-transfected HEK293 cells was determined by Annexin V/7-aminoactinomycin D (7AAD) double staining. Each bar graph represents mean data obtained from three independent experiments. (e) p53 target gene expression was measured by quantitative RT–PCR (qRT–PCR) in sihCdc73- and/or sip53-transfected HEK293 cells (left; each bar graph represents mean data from four independent experiments). Western blotting was performed to confirm the knockdown efficiency (right). (f,g) HCT116 p53-wt or p53-null cells were transfected with siCtrl or sihCdc73 for 48 h and were treated with the indicated dose of RITA for an additional 12 h. Apoptotic cells were quantitated by Annexin V/7AAD staining (f). qRT–PCR was performed to measureBAXgene expression (g). Each bar graph represents mean data from three independent experiments. (h) HCT116 p53-wt or p53-null cells stably expressing shCtrl or shhCdc73 were injected subcutaneously into nude mice. Thein vivogrowth of implanted HCT116 cells (5.0 × 106per nude mouse) was monitored (n=10). Error bars are presented as the mean±s.e.m. Statistical values were calculated using a two-tailedt-test (ns, not significant; *P<0.05; **P<0.01; ***P<0.001). 1a and Supplementary Table 1 ). Therefore, p53 expression was examined separately and it was confirmed that p53 mRNA and protein levels were increased in hCdc73-silenced HEK293 cells ( Fig. 1b and Supplementary Fig. 1g ) and HCT116 colon cancer cells ( Fig. 1c and Supplementary Fig. 1h,i ). Figure 1: hCdc73 controls apoptosis via p53. ( a ) The differential gene expression in siCtrl- versus sihCdc73-transfected HEK293 cells was analysed by microarray. Significantly affected pathways are listed. ( b ) HEK293 cells were transfected with siCtrl or sihCdc73, and p53 expression was analysed by western blotting (upper panel) and reverse transcriptase–PCR (RT–PCR) (bottom panel). ( c ) HEK293 and HCT116 cells were transfected with siCtrl or sihCdc73, and hCdc73 and p53 levels were evaluated by western blotting. ( d ) The apoptosis of sihCdc73- and/or sip53-transfected HEK293 cells was determined by Annexin V/7-aminoactinomycin D (7AAD) double staining. Each bar graph represents mean data obtained from three independent experiments. ( e ) p53 target gene expression was measured by quantitative RT–PCR (qRT–PCR) in sihCdc73- and/or sip53-transfected HEK293 cells (left; each bar graph represents mean data from four independent experiments). Western blotting was performed to confirm the knockdown efficiency (right). ( f , g ) HCT116 p53-wt or p53-null cells were transfected with siCtrl or sihCdc73 for 48 h and were treated with the indicated dose of RITA for an additional 12 h. Apoptotic cells were quantitated by Annexin V/7AAD staining ( f ). qRT–PCR was performed to measure BAX gene expression ( g ). Each bar graph represents mean data from three independent experiments. ( h ) HCT116 p53-wt or p53-null cells stably expressing shCtrl or shhCdc73 were injected subcutaneously into nude mice. The in vivo growth of implanted HCT116 cells (5.0 × 10 6 per nude mouse) was monitored ( n =10). Error bars are presented as the mean±s.e.m. Statistical values were calculated using a two-tailed t -test (ns, not significant; * P <0.05; ** P <0.01; *** P <0.001). Full size image When p53 was silenced, the apoptosis induced by hCdc73 deficiency was almost completely eliminated ( Fig. 1d ). The increased expression of p53 target genes, including PUMA, BAX , TP53I3 and 14-3-3σ , which occurred in response to hCdc73 knockdown was similarly inhibited by p53 silencing ( Fig. 1e ). To confirm the involvement of p53 in hCdc73-mediated apoptosis, hCdc73 was silenced in HCT116 p53-wt and p53-null cells, and apoptosis was examined. To induce p53-dependent apoptosis, the cells were treated with reactivation of p53 and induction of tumour cell apoptosis (RITA) [24] . RITA-induced apoptosis and BAX gene expression were further enhanced by hCdc73 silencing in p53-wt HCT116 cells but not in p53-null HCT116 cells ( Fig. 1f,g ). Together, these results implicated p53 in hCdc73-mediated apoptosis. To further investigate the potential link between hCdc73 and p53, we examined the effect of hCdc73 on the growth of solid tumours derived from p53-wt or p53-null HCT116 cells in nude mice ( Fig. 1h and Supplementary Fig. 1j,k ). Solid tumours derived from p53-wt cells exhibited slower growth when hCdc73 was silenced, while p53-null cells were not affected by hCdc73 silencing, indicating that hCdc73 controls cell growth in a p53-dependent manner. hCdc73 regulates mature p53 mRNA stability in the cytoplasm To understand how p53 levels were increased in hCdc73-deficient cells, we first examined whether hCdc73 repressed the transcription of p53, because it has been reported that PAFc represses immediate early genes and interleukin-1-inducible PLAU genes [25] . p53 gene transcription was active under basal conditions, and relatively strong RNA Pol II-Ser2P occupancy was detected at the coding region of the p53 locus in control cells ( Fig. 2a,b ). However, when hCdc73 expression was silenced, RNA Pol II-Ser2P occupancy was reduced and histone markers for active transcription—mono-ubiquitination of H2B on Lys120 residue and trimethylation of H3 on Lys4 residue [26] —were similarly diminished at p53 locus ( Fig. 2c,d ). As these results did not provide a logical explanation for the increased p53 expression in hCdc73-deficient cells, we next examined the post-transcriptional control of p53 expression. 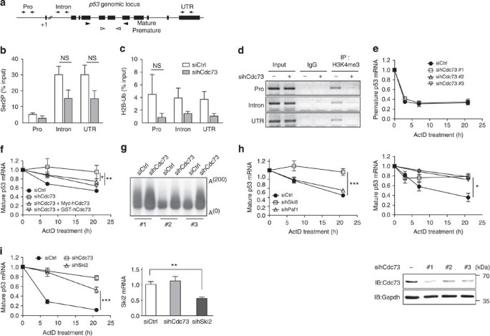Figure 2: hCdc73 controls mature p53 mRNA stability. (a) Schematic diagram of theTp53locus and the primers used for chromatin IP and reverse transcriptase–PCR (RT–PCR). (b–d) The chromatin occupancy of RNA Pol II with phosphorylated Ser2 on the C-terminal domain (CTD) (b), monoubiquitinated H2B (c) and trimethylated H3K4 (d) at theTp53locus was measured in siCtrl- or sihCdc73-transfected HEK293 cells. (e) The RNA stability of premature (upper panel) and mature (middle panel) p53 mRNA was measured by quantitative RT–PCR. The knockdown efficiency of each sihCdc73 construct was measured by western blotting (bottom panel). (f) Mature p53 mRNA stability was measured in sihCdc73-transfected HEK293 cells overexpressing Myc- or GST-hCdc73. (g) The poly(A) length on p53 mRNA was measured 60 h after transfection with siCtrl or sihCdc73. (h,i) The stability of mature p53 mRNA was determined in HEK293 cells transfected with the indicated short interfering RNAs. Each graph represents mean data from three independent experiments. Error bars are presented as the mean±s.e.m. Statistical values were calculated using a two-tailedt-test (ns, not significant; *P<0.05; **P<0.01; ***P<0.001). Figure 2: hCdc73 controls mature p53 mRNA stability. ( a ) Schematic diagram of the Tp53 locus and the primers used for chromatin IP and reverse transcriptase–PCR (RT–PCR). ( b – d ) The chromatin occupancy of RNA Pol II with phosphorylated Ser2 on the C-terminal domain (CTD) ( b ), monoubiquitinated H2B ( c ) and trimethylated H3K4 ( d ) at the Tp53 locus was measured in siCtrl- or sihCdc73-transfected HEK293 cells. ( e ) The RNA stability of premature (upper panel) and mature (middle panel) p53 mRNA was measured by quantitative RT–PCR. The knockdown efficiency of each sihCdc73 construct was measured by western blotting (bottom panel). ( f ) Mature p53 mRNA stability was measured in sihCdc73-transfected HEK293 cells overexpressing Myc- or GST-hCdc73. ( g ) The poly(A) length on p53 mRNA was measured 60 h after transfection with siCtrl or sihCdc73. ( h , i ) The stability of mature p53 mRNA was determined in HEK293 cells transfected with the indicated short interfering RNAs. Each graph represents mean data from three independent experiments. Error bars are presented as the mean±s.e.m. Statistical values were calculated using a two-tailed t -test (ns, not significant; * P <0.05; ** P <0.01; *** P <0.001). Full size image RNA stability was determined using primer sets specific to the premature and mature forms of p53 mRNA ( Fig. 2a ). The stability of mature p53 mRNA, but not premature mRNA, was significantly increased in hCdc73-deficient cells ( Fig. 2e ). To exclude off-target effects, three short interfering RNAs that target different regions of hCdc73 were tested. Mature p53 mRNA became unstable when hCdc73 was ectopically co-expressed in hCdc73-silenced cells ( Fig. 2f ). In accordance with increased mRNA stability, p53 mRNA was repeatedly observed with a longer poly(A) tail by hCdc73 knock down ( Fig. 2g ). In addition, although the stability of mature p53 mRNA remained unchanged in hPaf1-silenced cells, hSki2 or hSki8 deficiency resulted in a similar effect as hCdc73 silencing ( Fig. 2h,i and Supplementary Fig. 2a ). Therefore, p53 mRNA stability might be controlled by hCdc73 along with the SKI complex in a PAFc-independent manner. In contrast, p53 protein stability was not affected by hCdc73 silencing ( Supplementary Fig. 2b,c ). Cytoplasmic hCdc73 associates with p53 mRNA Using RNA separately isolated from the nucleus and the cytoplasm, the effect of hCdc73 on p53 mRNA stability was examined. The stability of cytoplasmic p53 mature mRNA was significantly enhanced by hCdc73 silencing, while it was indistinguishable for nuclear mRNA ( Fig. 3a ). As Cdc73 functionally interacts with 3′ mRNA processing factors [27] , we asked whether hCdc73 physically associated with mature p53 mRNA in the cytoplasm. The cytoplasmic fraction (S1) of HEK293 cells was prepared in polysome lysis buffer (PLB) ( Fig. 3b ) and hCdc73 binding to mature p53 mRNA was determined by RNA-immunoprecipitation (RNA-IP, see Methods) ( Fig. 3c,d and Supplementary Fig. 3a ). Physical association was observed between endogenous hCdc73 and processed mature p53 mRNA (p53-5′) but not premature p53 mRNA (p53-intron). In contrast, an interaction between endogenous hPaf1 and p53 mRNA was not detected with either premature or mature p53 mRNA, verifying that the regulation of p53 mRNA by hCdc73 is independent of the conventional PAFc. Physical interaction between the hSki8 and p53 mRNA was also confirmed ( Fig. 3e ), supporting the role of SKI complex in controlling the stability of p53 mRNA ( Fig. 2h,i ). We validated the specific interaction between hCdc73 and p53 mRNA using an in vitro -synthesized biotinylated p53 mRNA pull-down assay ( Fig. 3f ). Endogenous hCdc73 protein was specifically precipitated with the biotinylated p53 mRNA, because no binding occurred when excess non-biotinylated p53 mRNA was used as a competitor. A heterogeneous nuclear ribonucleoprotein Q, a known p53 mRNA-binding protein, was used as a positive control [28] . We then examined the region of p53 mRNA that hCdc73 binds. A series of p53 mRNA deletion constructs were generated and tested for hCdc73 interaction using the in vitro RNA pull-down assay ( Supplementary Fig. 3b ). A specific interaction with hCdc73 was observed only when the 5′-UTR region of p53 mRNAs was included in the construct. Although hCdc73 also associated with the coding DNA sequence (CDS) of p53 mRNA, their interaction was not inhibited by cold competitor, suggesting that this interaction was non-specific. Based on these results, we concluded that the interaction occurs through the 5′-UTR region of p53 mRNA. 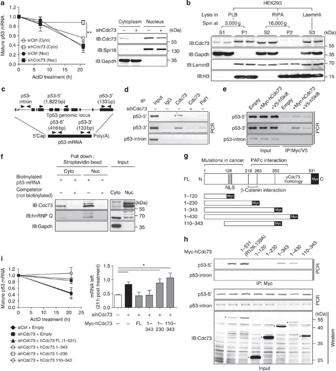Figure 3: hCdc73 associates with mature p53 mRNA. (a) Cytoplasmic and nuclear RNA from siCtrl- or sihCdc73-transfected HEK293 cells were assayed to determine p53 mRNA stability (left). The cellular fractionation was confirmed by western blotting with antibodies against Spt16 (nucleus) and GAPDH (cytoplasm) (right). (b) The cytoplasmic fraction (S1) was prepared in PLB buffer and analysed. For comparison, cells were lysed in three different lysis buffers (PLB, RIPA and Laemmli). Anti-GAPDH (cytoplasm) and anti-histone H3 (nucleus) antibodies were used to confirm the fractionation. (c) Schematic diagram of theTp53locus and the primers used for RNA-IP. (d) RNA-IP was performed in the S1 fraction from HEK293 cells using IgG, anti-Cdc73 and anti-Paf1 antibodies, and reverse transcriptase–PCR with the indicated primer sets. (e) Transfected HEK293 cells were subjected to RNA-IP using Myc or V5 antibodies. (f) The RNA pull-down assay was performed with the S1 fraction usingin vitrosynthesized and biotinylated p53 mRNA. (g) Schematic diagram of FL and truncated hCdc73. (h) HEK293 cells were transfected with the indicated plasmids and RNA-IPs were performed with an anti-Myc antibody (top). The expression of the transfected proteins was examined by western blotting for Cdc73 (bottom). The asterisks indicate FL or truncated hCdc73 protein. (i) HEK293 cells were transfected with the indicated short interfering RNAs and plasmids. The stability of mature p53 mRNA was measured after actinomycin D (ActD) treatment. The data are presented with a decay graph (left). In addition, the amounts of p53 mRNA present at 21 h post ActD treatment are shown in the bar graph (right). Each graph represents mean data from three independent experiments and error bars are presented as the mean±s.e.m. Statistical values were calculated using a two-tailedt-test (ns, not significant; *P<0.05; **P<0.01). Figure 3: hCdc73 associates with mature p53 mRNA. ( a ) Cytoplasmic and nuclear RNA from siCtrl- or sihCdc73-transfected HEK293 cells were assayed to determine p53 mRNA stability (left). The cellular fractionation was confirmed by western blotting with antibodies against Spt16 (nucleus) and GAPDH (cytoplasm) (right). ( b ) The cytoplasmic fraction (S1) was prepared in PLB buffer and analysed. For comparison, cells were lysed in three different lysis buffers (PLB, RIPA and Laemmli). Anti-GAPDH (cytoplasm) and anti-histone H3 (nucleus) antibodies were used to confirm the fractionation. ( c ) Schematic diagram of the Tp53 locus and the primers used for RNA-IP. ( d ) RNA-IP was performed in the S1 fraction from HEK293 cells using IgG, anti-Cdc73 and anti-Paf1 antibodies, and reverse transcriptase–PCR with the indicated primer sets. ( e ) Transfected HEK293 cells were subjected to RNA-IP using Myc or V5 antibodies. ( f ) The RNA pull-down assay was performed with the S1 fraction using in vitro synthesized and biotinylated p53 mRNA. ( g ) Schematic diagram of FL and truncated hCdc73. ( h ) HEK293 cells were transfected with the indicated plasmids and RNA-IPs were performed with an anti-Myc antibody (top). The expression of the transfected proteins was examined by western blotting for Cdc73 (bottom). The asterisks indicate FL or truncated hCdc73 protein. ( i ) HEK293 cells were transfected with the indicated short interfering RNAs and plasmids. The stability of mature p53 mRNA was measured after actinomycin D (ActD) treatment. The data are presented with a decay graph (left). In addition, the amounts of p53 mRNA present at 21 h post ActD treatment are shown in the bar graph (right). Each graph represents mean data from three independent experiments and error bars are presented as the mean±s.e.m. Statistical values were calculated using a two-tailed t -test (ns, not significant; * P <0.05; ** P <0.01). Full size image To identify the hCdc73 domain responsible for interacting with p53 mRNA, a series of hCdc73 deletion mutants was constructed ( Fig. 3g ). hCdc73 (531 amino acids) harbours a yCdc73 homology domain at the carboxy terminus. An internal domain (aa 227–413) near the C terminus of hCdc73 is required for interaction with PAFc [29] , [30] , whereas the β-catenin-interacting domain is located near the amino terminus [29] , [31] . To maintain the interaction with p53 mRNA, the N terminus region (aa 1–343) of hCdc73 was required ( Fig. 3h ); this region is enriched in the somatic and germline mutations observed in HPT-JT and parathyroid tumours [29] . A hCdc73 (R126/139A) mutant with a partial defect in nuclear localization ( Supplementary Fig. 3c and ref. 32 ) exhibited a stronger interaction with mature p53 mRNA, confirming that the p53 mRNA-hCdc73 interaction occurred in the cytoplasm. To investigate whether the p53 mRNA-hCdc73 interaction was necessary to control p53 mRNA stability, either full-length or mutant forms of hCdc73 were introduced into hCdc73-silenced cells, and mature p53 mRNA stability was measured ( Fig. 3i ). Reconstitution with hCdc73 FL or hCdc73 (1–343), both of which bind to p53 mRNA, reversed the increased p53 mRNA stability, while shorter forms were not. These data suggest that the mRNA-hCdc73 interaction was necessary for regulating p53 mRNA stability. hCdc73 physically interacts with eEF1Bγ to bind to p53 mRNA To understand how cytoplasmic hCdc73 controls p53 mRNA stability, cytoplasmic proteins that interact with hCdc73 were identified. The cytoplasmic fraction from GST-hCdc73-transfected HEK293 cells was analysed by glutathione S -transferase (GST) pull-down assays and mass spectrometry ( Fig. 4a ). Of the several hCdc73-binding candidates, Tsen54 (a component of the transfer RNA splicing complex) and eEF1Bγ (a component of the translation elongation complex) were selected for further validation based on their reported roles in RNA biology [33] , [34] . Physical interactions between hCdc73 and Tsen54 or eEF1Bγ were confirmed using ectopically expressed Myc-hCdc73 and eEF1Bγ ( Fig. 4b,c and Supplementary Fig. 4a,b ). Next, we examined the contributions of Tsen54 and eEF1Bγ to the regulation of p53 mRNA stability. eEF1Bγ silencing, but not Tsen54 silencing, significantly increased mature p53 mRNA stability similar to hCdc73-deficient cells, indicating that eEF1Bγ participates in the regulation of p53 mRNA stability ( Fig. 4d ). 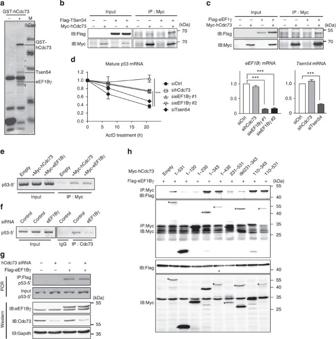Figure 4: eEF1Bγ, which interacts with cytoplasmic hCdc73, is required for the hCdc73-p53 mRNA association. (a) GST pull-down assays were performed in GST empty vector- or GST-hCdc73-transfected HEK293 cells and were analysed by silver staining. (b,c) The interactions between Myc-hCdc73 and FLAG-Tsen54 (b) or FLAG-eEF1Bγ (c) were analysed in transfected HEK293 cells. (d) Mature p53 mRNA stability was measured in HEK293 cells transfected with the indicated short interfering RNAs (siRNAs) (left). The knockdown efficiency of each siRNA was measured by quantitative reverse transcriptase–PCR (right). Each graph represents mean data from three independent experiments and error bars are presented as the mean±s.e.m. Statistical values were calculated using a two-tailedt-test (ns, not significant; ***P<0.001). (e–g) RNA-IPs were performed in HEK293 cytoplasmic lysates transfected with the indicated plasmids or siRNAs. (h) The interaction between hCdc73 and eEF1Bγ was analysed in HEK293 cells transfected with the indicated plasmids. Figure 4: eEF1Bγ, which interacts with cytoplasmic hCdc73, is required for the hCdc73-p53 mRNA association. ( a ) GST pull-down assays were performed in GST empty vector- or GST-hCdc73-transfected HEK293 cells and were analysed by silver staining. ( b , c ) The interactions between Myc-hCdc73 and FLAG-Tsen54 ( b ) or FLAG-eEF1Bγ ( c ) were analysed in transfected HEK293 cells. ( d ) Mature p53 mRNA stability was measured in HEK293 cells transfected with the indicated short interfering RNAs (siRNAs) (left). The knockdown efficiency of each siRNA was measured by quantitative reverse transcriptase–PCR (right). Each graph represents mean data from three independent experiments and error bars are presented as the mean±s.e.m. Statistical values were calculated using a two-tailed t -test (ns, not significant; *** P <0.001). ( e – g ) RNA-IPs were performed in HEK293 cytoplasmic lysates transfected with the indicated plasmids or siRNAs. ( h ) The interaction between hCdc73 and eEF1Bγ was analysed in HEK293 cells transfected with the indicated plasmids. Full size image Although eEF1Bγ is a structural component of the eukaryotic elongation complex (eEF1) that controls the transfer of aminoacyl tRNAs to ribosomes during translation, it is dispensable for translation [35] , [36] . Interestingly, eEF1Bγ was shown to have RNA-binding properties [34] , [37] . Therefore, we determined whether eEF1Bγ bound to mature p53 mRNA ( Fig. 4e ). Myc-eEF1Bγ bound to p53 mRNA to a comparable degree as did Myc-hCdc73. To evaluate the inter-dependency of hCdc73 and eEF1Bγ for binding to p53 mRNA, hCdc73 binding to p53 mRNA was measured in eEF1Bγ-silenced cells ( Fig. 4f ). hCdc73 failed to bind to p53 mRNA in eEF1Bγ-silenced cells, clearly suggesting that eEF1Bγ was necessary for hCdc73 binding to p53 mRNA. However, hCdc73 silencing did not affect eEF1Bγ binding to p53 mRNA ( Fig. 4g ). As a next, we performed IP assays using a series of hCdc73 deletion mutants and identified the hCdc73 domain that was required for interacting with eEF1Bγ ( Fig. 4h ). The minimum domain for eEF1Bγ binding spanned amino acids 110–343 of hCdc73, which partially overlaps with the p53 mRNA interaction domain. This domain was also responsible for the physical interaction between hCdc73 and hSki8 ( Supplementary Figs 4c,d ). These results suggested that the interaction between hCdc73 and eEF1Bγ was required for hCdc73 to bind to p53 mRNA. However, as the hCdc73 mutant (110–343) failed to regulate p53 mRNA stability in hCdc73-silenced cells ( Fig. 3i ), the physical interaction between hCdc73 and eEF1Bγ was required but was not sufficient to mediate the hCdc73-dependent regulation of p53 mRNA stability. Cytoplasmic hCdc73 forms a high-molecular-weight complex To understand the molecular architecture of cytoplasmic hCdc73-containing complexes, nuclear and cytoplasmic extracts were prepared from HEK293 cells and were fractionated by chromatography on a size-exclusion column ( Fig. 5a ). As previously reported [38] , [39] , hCdc73 forms a high-molecular-weight complex with hPaf1, hLeo1, hCtr9 and hSki8 in the nucleus. Notably, at least two different mobility forms of hCdc73 were observed. A fast-migrating form of hCdc73 exhibited a similar distribution as other PAFc components. In the cytoplasm, hCdc73 was found in a high-molecular-weight complex with eEF1Bγ and hSki8. To test whether hCdc73 associates with eEF1Bγ and hSki8 as a single complex, we performed a sequential pull-down assay ( Supplementary Fig. 5a ). Although hCdc73 was detected in the secondary immunoprecipitate, hSki8 was not present. Therefore, it is likely to be that there are distinct complexes present, which contain hCdc73-eEF1Bγ, hSki8-eEF1Bγ or hCdc73-hSki8, instead of hCdc73-eEF1Bγ-hSki8 as a single complex. However, it is still possible that there are transient hCdc73-eEF1Bγ-hSki8 interactions. Altogether, these data suggested that cytoplasmic hCdc73 formed a structurally distinct mega complex with different functions than nuclear hCdc73. 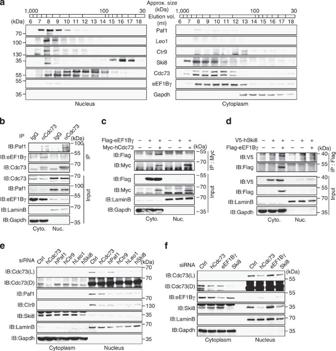Figure 5: hCdc73 forms a high-molecular-weight complex with eEF1Bγ and hSki8. (a) Fractionated cytoplasmic and nuclear extracts were analysed by western blotting with the indicated antibodies. The approximate sizes were estimated based on the elution profile of standard proteins. (b,c) Cytoplasmic and nuclear fractions were subjected to immunoprecipitation. Interactions between endogenous (b) and exogenous (c) proteins were examined by immunoprecipitation with anti-Cdc73 and anti-Myc antibodies, respectively. (d) HEK293 cells were transfected with V5-hSki8 and FLAG-eEF1Bγ, and the cytoplasmic and nuclear fractions were immunoprecipitated with an anti-FLAG antibody. (e,f) HEK293 cells were transfected with the indicated short interfering RNAs, and the cytoplasmic and nuclear fractions were subjected to western blotting with the indicated antibodies. Figure 5: hCdc73 forms a high-molecular-weight complex with eEF1Bγ and hSki8. ( a ) Fractionated cytoplasmic and nuclear extracts were analysed by western blotting with the indicated antibodies. The approximate sizes were estimated based on the elution profile of standard proteins. ( b , c ) Cytoplasmic and nuclear fractions were subjected to immunoprecipitation. Interactions between endogenous ( b ) and exogenous ( c ) proteins were examined by immunoprecipitation with anti-Cdc73 and anti-Myc antibodies, respectively. ( d ) HEK293 cells were transfected with V5-hSki8 and FLAG-eEF1Bγ, and the cytoplasmic and nuclear fractions were immunoprecipitated with an anti-FLAG antibody. ( e , f ) HEK293 cells were transfected with the indicated short interfering RNAs, and the cytoplasmic and nuclear fractions were subjected to western blotting with the indicated antibodies. Full size image To confirm the physical interaction between cytoplasmic hCdc73 and eEF1Bγ, cytoplasmic and nuclear fractions were prepared, and IP assays against endogenous hCdc73 or ectopically expressed Myc-hCdc73 were performed ( Fig. 5b,c ). Endogenous eEF1Bγ and ectopically expressed Flag-eEF1Bγ were predominantly expressed in the cytoplasm, and as a result the physical interaction between hCdc73 and eEF1Bγ was only detected in the cytoplasm. Similarly, the physical interaction between eEF1Bγ and hSki8 was only observed in the cytoplasm ( Fig. 5d ). These data confirmed that hCdc73 formed a distinct complex with eEF1Bγ and hSki8 in the cytoplasm. When hCtr9 or hLeo1 is silenced, other PAFc components are similarly downregulated, indicating that the stoichiometry of the PAFc is intimately linked to protein level control [15] . As has been reported, hCdc73 was downregulated in the nucleus of hCtr9- or hLeo1-deficient cells ( Fig. 5e ). However, cytoplasmic hCdc73 levels were not affected in these cells, confirming that cytoplasmic hCdc73 is independent of the conventional PAFc. Nuclear and cytoplasmic hCdc73 levels were reduced to a similar extent in hSki8-silenced cells ( Fig. 5e ). Therefore, we wondered whether the protein levels of cytoplasmic hCdc73 were regulated by the levels of eEF1Bγ and hSki8. As expected, the cytoplasmic, but not nuclear, levels of hCdc73 were decreased in eEF1Bγ-silenced cells ( Fig. 5f ), confirming that cytoplasmic hCdc73 forms a functional complex with eEF1Bγ, and that its activity as well as its structural integrity are tightly controlled by hSki8 and eEF1Bγ. Cytoplasmic hCdc73 involved in p53-dependent carcinogenesis The p53 tumour suppressor plays essential roles in the maintenance of genomic stability under DNA-damaging conditions [1] . Although the steady-state protein levels of p53 are low, p53 protein is stabilized and hyperactivated under stress conditions such that p53 undergoes homeostatic regulation on demand. We ascertained whether the expression or the activity of cytoplasmic hCdc73 was altered during the DNA damage response. To induce DNA damage and activate p53, we treated cells with RITA, fluorouracil (5-FU) and doxorubicin (Doxo). We then examined hCdc73 protein levels in the fractionated nuclear and cytoplasmic extracts ( Fig. 6a ). The cytoplasmic hCdc73 levels dramatically decreased and nuclear p53 protein levels increased following treatment with the conventional genotoxic drugs 5-FU and Doxo. However, hCdc73 levels were not dramatically changed by RITA. Although RITA induces p53 activation and Chk-1- and Chk-2-dependent DNA damage response, its mode of action differs from 5-FU and Doxo that directly cause DNA damage via intercalation [24] , [40] , [41] . This result indicated that certain DNA stress agents, such as 5-FU and Doxo, specifically affect cytoplasmic hCdc73 levels. 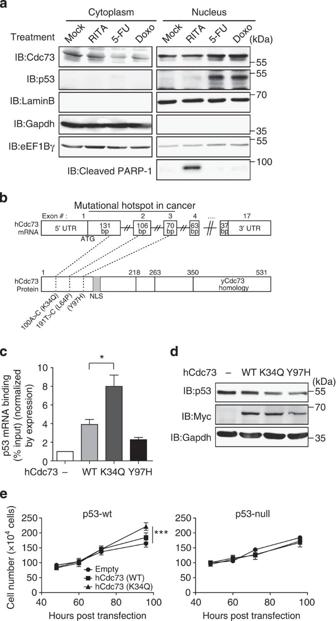Figure 6: Mutations in hCdc73 affect p53 levels. (a) HCT116 cells were treated with RITA (10 nM), 5-FU (10 μg ml−1), or Doxo (50 nM) for 4 h. The cytoplasmic and nuclear fractions were analysed by western blotting with the indicated antibodies. (b) Schematic diagram of hCdc73 highlighting the point mutations that have been observed in cancer patients. (c) RNA-IP of hCdc73 in the cytoplasmic lysate of transfected HEK293 cells, followed by quantitative reverse transcriptase–PCR. (d) Endogenous p53 levels were measured by western blotting in wild-type (WT) or mutant Myc-hCdc73-transfected HEK293 cells. (e) HEK293 (1 × 105) cells were transfected with the indicated plasmids and cultured for up to 96 h. The viable cells were counted using a haemocytometer at the indicated time points. Each graph represents mean data from three independent experiments and error bars are presented as the mean±s.e.m. Statistical values were calculated using a two-tailedt-test (ns, not significant; *P<0.05; ***P<0.001). Figure 6: Mutations in hCdc73 affect p53 levels. ( a ) HCT116 cells were treated with RITA (10 nM), 5-FU (10 μg ml −1 ), or Doxo (50 nM) for 4 h. The cytoplasmic and nuclear fractions were analysed by western blotting with the indicated antibodies. ( b ) Schematic diagram of hCdc73 highlighting the point mutations that have been observed in cancer patients. ( c ) RNA-IP of hCdc73 in the cytoplasmic lysate of transfected HEK293 cells, followed by quantitative reverse transcriptase–PCR. ( d ) Endogenous p53 levels were measured by western blotting in wild-type (WT) or mutant Myc-hCdc73-transfected HEK293 cells. ( e ) HEK293 (1 × 10 5 ) cells were transfected with the indicated plasmids and cultured for up to 96 h. The viable cells were counted using a haemocytometer at the indicated time points. Each graph represents mean data from three independent experiments and error bars are presented as the mean±s.e.m. Statistical values were calculated using a two-tailed t -test (ns, not significant; * P <0.05; *** P <0.001). Full size image We next asked the effect of the somatic and germline mutations in hCdc73 that have been reported in parathyroid tumours on the regulation of p53. Most of the reported hCdc73 mutations in cancer are overrepresented in the N-terminal region [29] and hence we selected three missense mutations (K34Q, L64P and Y97H) ( Fig. 6b ). We eventually excluded the L64P mutation from our analysis, because this mutant failed to express comparable hCdc73 protein levels. Compared with wild-type hCdc73, the hCdc73 K34Q mutant exhibited stronger binding to p53 mRNA and interaction with eEF1Bγ protein ( Fig. 6c and Supplementary Fig. 5b ). hCdc73 K34Q is a gain-of-function mutant and overexpression of hCdc73 K34Q in the presence of endogenous hCdc73 reduced the steady-state levels of endogenous p53 protein ( Fig. 6d ). In addition, overexpressed hCdc73 K34Q accelerated the growth of HCT116 p53-wt cells but not HCT116 p53-null cells ( Fig. 6e ). Although the hCdc73 K34Q mutant explained the role of hCdc73-p53 mRNA associations and its contribution to the p53-mediated carcinogenesis, the cancer-driven mutation Y97H did not. Overexpression of the hCdc73 Y97H mutant reduced endogenous p53 levels, but its binding to p53 mRNA was not enhanced ( Fig. 6c,d ). Our data indicates that hCdc73 indeed affects p53 mRNA and p53-mediated apoptosis. However, as the results carried out by two independent point mutations were not consistent, it is premature to conclude that alternations in hCdc73-p53 mRNA interaction directly contribute to carcinogenesis in parathyroid carcinoma and HPT-JT syndrome. In this report, we demonstrated that cytoplasmic hCdc73 bound to and destabilized mature p53 mRNA, thereby controlling endogenous p53 levels and p53-mediated apoptosis. Under basal conditions, the steady-state levels of mature p53 mRNA was controlled by the cytoplasmic hCdc73-eEF1Bγ complex that bound to and degraded p53 mRNA ( Fig. 7a ). Under genotoxic stress conditions, the transient shortage of cytoplasmic hCdc73 released mature p53 mRNA, increasing p53 expression on demand ( Fig. 7b ). In contrast, mutations in hCdc73 that affect the binding affinity to p53 mRNA might provide a selective advantage for cell growth, as evidenced by the hCdc73 K34Q mutant found in parathyroid tumours ( Fig. 7c ). 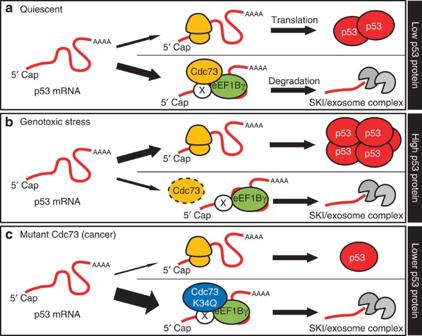Figure 7: Working hypothesis of cytoplasmic hCdc73-mediated p53 regulation. (a) Under quiescent conditions, the steady-state level of p53 mRNA is controlled by hCdc73-eEF1Bγ. (b) In response to genotoxic stress, the decrease in cytoplasmic hCdc73 transiently enhances p53 levels. (c) Mutations in hCdc73 (for example, K34Q) result in a tighter association with p53 mRNA, leading to p53 misregulation. Figure 7: Working hypothesis of cytoplasmic hCdc73-mediated p53 regulation. ( a ) Under quiescent conditions, the steady-state level of p53 mRNA is controlled by hCdc73-eEF1Bγ. ( b ) In response to genotoxic stress, the decrease in cytoplasmic hCdc73 transiently enhances p53 levels. ( c ) Mutations in hCdc73 (for example, K34Q) result in a tighter association with p53 mRNA, leading to p53 misregulation. Full size image hCdc73 is a component of the PAFc, which mainly functions in the nucleus with RNA polymerase II (ref. 11 ). We also observed that hCdc73 is mainly localized in the nucleus ( Supplementary Fig. 3c ). However, we demonstrated that a minor fraction of hCdc73 was also present and functional in high-molecular-weight complexes in the cytoplasm. The molecular composition and the function of the nuclear and cytoplasmic complexes harbouring hCdc73 were distinct. The majority of hCdc73 localizes in the nucleus and is associated with the PAFc and hCtr9, hPaf1, hLeo1 and hSki8 to control transcription [10] . In the cytoplasm, only a minor fraction of hCdc73 is available for interaction with eEF1Bγ and hSki8 to control RNA stability. Currently, it is not clear what controls the formation of the distinct hCdc73 complexes or what transports hCdc73 between the nuclear and cytoplasmic compartments. Recently, actinin 2 and 3 have been proposed to induce the cytoplasmic accumulation of hCdc73 (ref. 42 ), implying that the cytoplasmic localization of hCdc73 might be actively regulated. In mammals, the SKI complex is composed of hSki2/hMtr4, hSki3 and hSki8, and participates in exosome-mediated RNA degradation [43] , [44] . We presented multiple lines of evidence suggesting that hCdc73 cooperates with the SKI complex, along with eEF1Bγ, to regulate p53 mRNA stability in the cytoplasm. Previous study revealed eEF1A, which forms a functional complex with eEF1Bγ, has extensive homology with yeast Ski7p (24.8% sequence identity over a 210-aa region), which is required for the proper recruitment and activation of the SKI/Exosome complex during nonsense-mediated decay [45] . Altogether, these imply that eEF1Bγ may functionally interact with the SKI/Exosome complex, along with cytoplasmic hCdc73, to provide quality control of mature p53 mRNA. We showed that eEF1Bγ binds to p53 mRNA and this interaction was essential for the interaction between hCdc73 and p53 mRNA. Thus, hCdc73 interaction with p53 mRNA occurs via eEF1Bγ. We also showed that hSki8 controls p53 mRNA stability. As it is well known that hSki8 interacts with hCdc73 (ref. 15 ), p53 mRNA degradation via the SKI complex might require hCdc73 interaction with hSki8. Based on the observation that hCdc73 interacts with both eEF1Bγ and hSki8, we speculated that hCdc73 functions to link the mRNA-eEF1Bγ and the SKI (RNA degradation) complex. Although eEF1Bγ is commonly considered to be a structural component of the translation elongation complex (eEFs) [36] , we show that eEF1Bγ also serves as a binding platform for hCdc73 to bind p53 mRNA. In the recently published proteomics study using artificial pre-mRNAs, hCdc73 and eEF1Bγ were co-purified with 3′-pre-mRNA-processing complexes in humans [37] . Moreover, eEF1Bγ was co-purified with other translation factors. Therefore, it will be interesting to consider the functional and physical cross-talk between RNA processing and translation control via hCdc73. Both the quality and the turnover of mature mRNA are tightly controlled by 3′–5′ RNA exosome and by 5′–3′ exonucleases in the cytoplasm [44] . Regulated mRNAs harbour unique molecular signatures, including translational abnormalities, short poly(A) tails, or RNA sequences that recruit RNA decay enzymes [46] . Although we demonstrated that cytoplasmic hCdc73 bound to p53 mRNA and induced its degradation, we do not know whether it controls p53 mRNA quality or mature p53 mRNA turnover. To answer this, it will be critical to identify the RNA signatures that are essential for mediating the interaction between p53 mRNA and cytoplasmic hCdc73. In this study, we showed that hCdc73 associates with the 5′-UTR region of p53 mRNA ( Supplementary Fig. 3b ). Therefore, we postulate that RNA structures or abnormalities in the 5′-UTR of p53 mRNA might be the target for interaction. Interestingly, similar to eEF1Bγ, proteins in the translation machinery such as RPL26 and nucleolin bind the 5′-UTR of p53 mRNA and control its mRNA levels [47] . However, more in-depth studies are necessary to uncover the molecular mechanism that controls the specific interactions between hCdc73 and target mRNA. Although we demonstrated the inhibitory effect of hCdc73 on p53, hCdc73 was initially proposed as a tumour suppressor. The overexpression of hCdc73 reduces cell proliferation in vitro and reduced hCdc73 levels are observed in human tumour tissues [21] , [48] . We propose three points to consider when interpreting this somewhat contradictory result. First, many in vitro studies analysing the molecular function of hCdc73 used HeLa cells, which express SV40 large T antigen (SV40LT) [32] , [38] , [48] . SV40LT destabilizes p53; hence, the effect of hCdc73 on p53 might be masked in HeLa cells. In addition, Iwata et al. [23] showed the effect of hCdc73 on cell proliferation changed in response to expression status of SV40LT. Second, Cdc73-deficient mouse embryonic fibroblast cells exhibited massive apoptosis, which cannot be explained if Cdc73 is a mere tumour suppressor [22] . Finally, most of the previous immunohistochemistry studies focused on nuclear hCdc73 and neglected the contribution of cytoplasmic hCdc73 (refs 21 , 49 ). It was especially encouraging to identify hCdc73 mutations that affect cellular levels of p53 in tissues from cancer patients ( Fig. 6d ). The single point mutation K34Q in eEF1Bγ- and the mRNA-binding domain of hCdc73 lowered steady-state levels of p53 proteins and exhibited strong binding ability to p53 mRNA ( Fig. 6c,d ). This result indicates that hCdc73-p53 mRNA association is a critical step in controlling p53. However, other cancer-driven hCdc73 mutations, such as Y97H, exhibited different effects. The overexpression of this mutant also lowered endogenous p53 levels, but it was not due to increased association with p53 mRNA. Therefore, this result indicates that hCdc73 controls p53 levels by additional methods. If other processes such as cellular localization or binding to the RNA degradation complex are altered, it could affect cytoplasmic function of hCdc73. Recently, the L95P mutation in hCdc73 was reported to disrupt the nucleolar localization of hCdc73 and to cause HPT-JT syndrome [50] , confirming that misregulation of the cellular localization of hCdc73 may contribute to carcinogenesis. In this work, we elucidated the mRNA-binding domain of hCdc73 and a target site that can enhance their binding affinity. Therefore, therapeutic peptides that compete tumorigenic hCdc73 binding to p53 mRNA can be considered. Moreover, it will be essential to understand the diverse mechanistic aspects of the interaction between hCdc73 and p53 mRNA, and how misregulation of this interaction contributes to cancer. Cells and reagents HEK293 (obtained from ATCC, Manassas, VA) and HCT116 (kind gift from Dr Bert Vogelstein, Johns Hopkins University, Baltimore, MD) cells were maintained in DMEM (Welgene, Korea) supplemented with 10% fetal bovine serum (Hyclone, Logan, UT) and 1% penicillin/streptomycin (Invitrogen, Carlsbad, CA). In most of transfection experiment, cells were incubated with Lipofectamin 2000 (Invitrogen) for 48 h before analysis. Doxo, 5-FU and actinomycin D were purchased from Sigma (St Louis, MO, USA). RITA was purchased from Santa Cruz Biotechnology (Santa Cruz, CA). Plasmids and short hairpin RNA Myc-hCdc73 has been described previously [51] . To create GST-hCdc73, hCdc73 was subcloned into the pEBG vector. To make mutant Myc-hCdc73, site-directed mutagenesis was performed. For FLAG-eEF1Bγ and FLAG-Tsen54, HEK293 complementary DNA was PCR amplified and cloned into pFLAG-CMV. To create pSK-p53(FL), p53 cDNA, including the CDS, 5′-UTR and 3′-UTR, was cloned into pBluescript SK(−) (Clontech Takara Bio, Japan). Sequence information on the PCR primers and synthetic oligomers used in this study are provided in Supplementary Table 2 . IP and immunoblotting The cells were lysed in lysis buffer (150 mM NaCl, 25 mM Tris–HCl, pH 7.4, 1% Triton X-100, 0.5% Deoxycholic acid, 0.1% SDS) supplemented with protease inhibitors. Total lysates (1 mg) were incubated with 2 μg of primary antibody along with Protein A/G agarose beads (Calbiochem, San Diego, CA). For input, 25 μg of each lysate was used. Polyclonal antibodies against Cdc73, Paf1, Ctr9 and Leo1 were purchased from Bethyl Laboratories (Montgomery, TX). For immunoblotting, anti-Cdc73 (1:1,000), anti-Myc (1:1,000) and anti-eEF1Bγ (1:2,000) monoclonal antibodies and rabbit polyclonal anti-FLAG (1:2,000) antibodies were purchased from Santa Cruz Biotechnology, and anti-Ski8 (1:2,000) antibody was purchased from Abnova (Taipei, Taiwan). Uncropped versions of the important immunoblottings are provided in Supplementary Fig. 6 . Chromatin IP Chromatin IP was performed as described previously with some modifications [25] . Briefly, 4 × 10 7 cells were cross-linked with 1% formaldehyde and lysed in cell lysis buffer (20 mM Tris–HCl, pH 8.0, 85 mM KCl, 0.5% NP-40, with protease inhibitors). Nuclear pellets were resuspended in nuclear lysis buffer (50 mM HEPES-KOH, pH 7.4, 140 mM NaCl, 1 mM EDTA, 1% Triton X-100, 0.1% sodium deoxycholate, with protease inhibitors) and sonicated using a Vibra-Cell sonicator. Cleared lysates were subjected to IP using 4 μg of the indicated antibodies with protein A/G agarose beads. DNA was eluted and purified using a PCR purification kit (NucleoGen, Korea). The PCR primer sequences are provided in Supplementary Table 2 . The data were normalized to the input signal. RNA isolation and real-time reverse transcriptase–PCR Total RNA was extracted using RNAiso plus (Takara Bio, Japan). RNA (1 μg) was reverse transcribed with ImProm-II Reverse Transcriptase (Promega, Madison, WI) using oligo(dT) or random primers (Promega). PCR analysis of the cDNA was performed on a StepOne Plus Real-Time PCR System (Applied Biosystems, Foster City, CA). In most of the PCR reactions, β-actin was used as the internal control. For mRNA stability measurement, 18s rRNA or 28s rRNA were used as the internal control. Cytoplasmic and nuclear RNA samples were prepared as previously described [52] . Briefly, cells were swelled in RSB (10 mM Tris–HCl, pH 7.4, 10 mM NaCl and 3 mM MgCl 2 ) and lysed in RSBG40 buffer (10 mM Tris–HCl, pH 7.4, 10 mM NaCl, 2 mM MgCl 2 , 10% glycerol, 0.5% NP-40, 0.5 mM dithiothreitol and 100 U ml −1 RNAseOUT). After centrifugation at 4,500 g , RNA was isolated separately from the cytoplasmic (supernatant) and nuclear (pellet) fractions. Microarray Total RNA was purified with an RNeasy Kit (Qiagen, Valencia, CA) and was amplified using a TotalPrep RNA Amplification Kit (Ambion, Austin, TX). cDNA was hybridized onto a HumanHT-12 V3 Expression BeadChip and was analysed using an Illumina BeadArray Reader (Illumina Inc., San Diego, CA). RNA immunoprecipitation RNA-IPs were performed as previously described [53] . Approximately 5 × 10 7 cells were lysed in PLB (100 mM KCl, 5 mM MgCl 2 , 10 mM HEPES, pH 7.0, and 0.5% Nonidet P-40) supplemented with protease inhibitors and 100 U ml −1 RNAse inhibitor. After centrifuging at 3,000 g , the supernatant was pre-cleared and then incubated with the indicated antibodies and protein A/G agarose beads for 4 h at 4 °C. After 6 washes with 0.5 ml PLB, the bound complexes were eluted in PLB buffer with 0.1% SDS and 300 μg ml −1 Proteinase K (Roche). RNA from the eluate was isolated using RNAiso Plus. RNA pull-down assay Streptavidin–biotin RNA pull-down assays were performed as previously described, with certain modifications [54] . Linearized pSK-p53(FL), pSK-p53(del3′), pSK-p53(del5′) or pSK-p53(CDS) were in vitro transcribed using T7 polymerase (Promega) and biotin-UTP (Roche). Biotinylated RNA (10 μg) was purified and incubated with 500 μg of cytoplasmic/nuclear extract in the presence of incubation buffer (20 mM Tris-Cl, pH 7.5, 50 mM NaCl, 2 mM MgCl 2 and 1% Tween-20) supplemented with protease inhibitors and 100 U ml −1 RNAse inhibitor. Streptavidin agarose resin (Pierce) was incubated at 4 °C for 4 h. Resin-bound proteins were eluted and subjected to western blotting. Apoptosis assay To measure apoptosis, 1 × 10 5 cells were stained with fluorescein isothiocyanate–Annexin V, propidium iodide (Sigma) or 7-aminoactinomycin D (Sigma) in 10 mM HEPES, pH 7.4, 140 mM NaCl and 2.5 mM CaCl 2 for 20 min at room temperature. The cells were analysed on a FACS Calibur flow cytometer (BD Biosciences). Cellular fractionation For the cytoplasmic and nuclear fractionation, 5 × 10 6 cells were resuspended in sucrose buffer (320 mM sucrose, 10 mM Tris–HCl, pH 8.0, 3 mM CaCl 2 , 2 mM MgOAc, 0.1 mM EDTA, 0.5% NP-40, 1 mM dithiothreitol and 0.5 mM phenylmethyl sulphonyl fluoride). After centrifugation at 600 g , the cytoplasmic (supernatant) fraction was removed. The pellet was washed with sucrose buffer without NP-40 and lysed in lysis buffer. The mixture was incubated on ice for 30 min and centrifuged at 13,000 g . The supernatant, which contained the soluble nuclear proteins, was removed. Size-exclusion chromatography The salt concentration of the cytoplasmic fraction was adjusted with 5 M NaCl, and this fraction was loaded onto a Superdex 200 10/300 GL Column (GE Healthcare Biosciences, Piscataway, NJ). The flow rate was 0.5 ml min −1 and 0.5 ml fractions were collected. Aldolase (158 kDa) and thyroglobulin (669 kDa) (GE Healthcare) were used for calibration. Stable cell line generation and solid tumour model Linearized hCdc73 short hairpin RNA expression constructs ( Supplementary Table 2 ) were transfected into HCT116 (p53-wt or p53-null) cells, which were then selected with puromycin (10 μg ml −1 ). Eight-week-old male BALB/c nude mice were used for the tumour xenograft model. Cells (5 × 10 6 ) were subcutaneously implanted in the dorsal flank. At least ten mice per group were included in each experiment. Tumour growth was measured using digital calipers twice a week, and the tumour volume was calculated as the (width 2 ) × (length) × 0.5 (ref. 55 ). All the experimental animal protocols were approved by the Institutional Animal Care and Use Committee of Seoul National University Hospital. GST pull-down and mass spectrometry analysis GST-hCdc73 or GST-empty construct was transfected to HEK293 cells and the cells were subsequently lysed in PLB. Lysates (10 mg) were incubated with glutathione sepharose 4B beads (GE Healthcare) at 4 °C for 4 h. After washing with PLB, the eluates were resolved by SDS–PAGE and stained using the PlusOne Silver Staining kit (GE Healthcare). The bands were excised and subjected to mass spectrometry analysis. Immunohistochemistry Cellular levels of p53 and caspase-3 proteins were measured on formalin-fixed, paraffin-embedded sections obtained from tumour-bearing Balb/c mice. Sections were blocked with normal goat serum (1:30, S2000, Vector Lab) and treated with primary anti-p53 antibody (1:200, OP43, Oncogene) or with primary anti-caspase-3 antibody (1:300, Abcam, ab13847) overnight at 4 °C. Following several washes, anti-mouse-IgG (1:250, BA9200, Vector Labs) or anti-rabbit-IgG (1:250, BA1100, Vector Labs) were used as secondary antibody. Sections were counterstained with Harris haematoxylin solution (HHS32, Sigma-Aldrich). Accession codes: Data are available in Gene Expression Omnibus (GEO; GSE61601 ). How to cite this article: Jo, J.-H. et al. Cytoplasmic parafibromin/hCdc73 targets and destabilizes p53 mRNA to control p53 mediated apoptosis. Nat. Commun. 5:5433 doi: 10.1038/ncomms6433 (2014).